Engineering thermal conductance using a two-dimensional phononic crystal Controlling thermal transport has become relevant in recent years. Traditionally, this control has been achieved by tuning the scattering of phonons by including various types of scattering centres in the material (nanoparticles, impurities, etc). Here we take another approach and demonstrate that one can also use coherent band structure effects to control phonon thermal conductance, with the help of periodically nanostructured phononic crystals. We perform the experiments at low temperatures below 1 K, which not only leads to negligible bulk phonon scattering, but also increases the wavelength of the dominant thermal phonons by more than two orders of magnitude compared to room temperature. Thus, phononic crystals with lattice constants ≥1 μm are shown to strongly reduce the thermal conduction. The observed effect is in quantitative agreement with the theoretical calculation presented, which accurately determined the ballistic thermal conductance in a phononic crystal device. Controlling thermal transport has become more relevant in recent years, in light of the strong push to develop novel energy harvesting techniques based on thermoelectricity [1] , the need to improve the heat dissipation out of semiconductor devices, and the push to increase the sensitivity of bolometric radiation detectors [2] . Traditionally, reduction of thermal conductivity is achieved by means including impurities, nanoparticles, voids, etc., which increase the scattering of the relevant energy carrying quanta, electrons and phonons. As the phonon thermal transport component is present in all conducting and insulating materials, a lot of research has lately focused on lowering phonon thermal conductivity using nanoscale structuring of materials [3] to increase scattering, with good results in improving thermoelectric materials [4] , for example. On the other hand, much less attention has been given to controlling phonon thermal conductance by engineering the phonon dispersion relations, in other words the phonon ‘band structure’. This could be achieved with the help of periodic phononic crystal (PnC) structures. Phononic crystals are the elastic analogues of the better known photonic crystals [5] , and are attractive from the point of view of manipulating the flow of vibrational energy, that is, sound and/or heat. The main feature of PnCs is the appearance of complete band gaps for certain frequencies in some cases, and a strong modification of the phononic band structure due to Bragg’s interference [6] , [7] . Early experimental studies on PnCs were restricted to macroscopic systems with millimeter-scale periodic structures, where sonic or ultrasonic waves in sub-MHz frequency range play a major role, and applications were typically limited to acoustic filtering, wave-guiding or focusing, for example [8] , [9] . Recent progress in nanofabrication technologies, however, enables us to create micro- and nano-scale periodic structures as small as the characteristic wavelength of GHz-frequency hypersonic waves [10] , [11] , allowing applications in RF communication technologies [12] and optomechanics [13] , as well. More interestingly for the topic here, GHz-frequency acoustic waves are nothing but a coherent collection of GHz phonons, and at sub-Kelvin temperatures, GHz phonons are the dominant thermal excitations. Thus, strong manipulation of thermal properties, such as thermal conduction and heat capacity, seems possible. Indeed, there are already a few reports of successful reduction of the room temperature thermal conductivity using periodic structures [14] , [15] , [16] , and some of the observed reduction was tentatively ascribed to coherent band stucture effects. However, in the room temperature studies, the dominant thermal phonons are really in the THz frequency range [17] , [18] , and no fully conclusive evidence on the coherent effects has been shown up-to-date. Here, we demonstrate both experimentally and theoretically that one can use coherent band structure effects to control phonon thermal conductance, with the help of periodically nanostructured PnCs. We have perforated suspended silicon nitride (SiN) membranes into square arrays of circular holes, to obtain two-dimensional PnCs ( Fig. 1 ). Two different lattice constants were used: one designed to have a complete phononic band gap at the characteristic energy of thermal dominant phonons at 0.1 K, and the other with no band gap. The membrane thickness and the hole-filling factor were the same for both structures, thus, a bulk phonon scattering model would predict identical thermal conductances. However, a large difference was seen in the experiment, fully explained by the difference in the band structures of the two samples. Moreover, for both samples the observed reduction of thermal conductance (as compared to an unperforated membrane) is in quantitative agreement with our ballistic thermal conductance calculation. 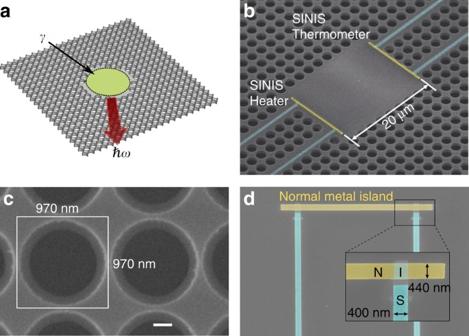Figure 1: The 2D membrane PnC device. (a) Schematic representation of a perforated membrane PnC geometry with a square array of circular holes, fabricated by e-beam lithography. The central region has a heater, which emits thermal phonons into the PnC structure. (b) A false colour scanning electron micrograph (s.e.m.) of the central region of the larger perioda=2425, nm PnC sample. The blue (Al) and yellow (Cu) lines are the metallic wiring which form the heater and thermometer elements at the centre of the PnC. The shorter period sample has the same wiring locations and dimensions. The full size of the perforated membrane is 100 μm × 100 μm. (c) A scanning electron micrograph of a region of the shorter period sample (black areas, empty space, grey areas SiN membrane), showing the unit cell size 970 nm × 970 nm and the width of the narrowest region ~60 nm. The sidewalls have a slight angle so that the bottom end of the hole is slightly smaller. Scale bar has length 200 nm. (d) A false colour s.e.m. of the heater/thermometer structure, consisting of a Cu normal metal wire (yellow) sandwiched between two normal metal-insulator-superconductor (NIS) tunnel junctions, connected to the measurement circuit by superconducting Al leads (blue). Figure 1: The 2D membrane PnC device. ( a ) Schematic representation of a perforated membrane PnC geometry with a square array of circular holes, fabricated by e-beam lithography. The central region has a heater, which emits thermal phonons into the PnC structure. ( b ) A false colour scanning electron micrograph (s.e.m.) of the central region of the larger period a =2425, nm PnC sample. The blue (Al) and yellow (Cu) lines are the metallic wiring which form the heater and thermometer elements at the centre of the PnC. The shorter period sample has the same wiring locations and dimensions. The full size of the perforated membrane is 100 μm × 100 μm. ( c ) A scanning electron micrograph of a region of the shorter period sample (black areas, empty space, grey areas SiN membrane), showing the unit cell size 970 nm × 970 nm and the width of the narrowest region ~60 nm. The sidewalls have a slight angle so that the bottom end of the hole is slightly smaller. Scale bar has length 200 nm. ( d ) A false colour s.e.m. of the heater/thermometer structure, consisting of a Cu normal metal wire (yellow) sandwiched between two normal metal-insulator-superconductor (NIS) tunnel junctions, connected to the measurement circuit by superconducting Al leads (blue). Full size image Design of the PnC device The square array was chosen for simplicity, and the circular hole shape to reduce the possibility of a mechanical weak point, such as a sharp corner, for cracking. Suspended SiN membranes and beams are widely used for micro- and nano-electromechanical devices [19] , [20] , [21] , [22] owing to their mechanical strength, stiffness and ease of processing. In addition, they are also used for low-temperature bolometric radiation detectors [23] , [24] and tunnel junction coolers [24] , [25] , [26] , [27] as a controllable, well-defined thermal link to the heat bath. (A famous example of this application is the Planck’s satellite high-frequency instrument [28] measuring the cosmic microwave background.) However, due to the strong suppression of bulk scattering of phonons in insulators at sub-K temperatures [29] , [30] , thermal phonons travel ballistically for very long distances, with mean free paths up to ~10 cm in polished crystalline Si samples [30] . In SiN at around 0.1 K, ballistic transport has also been observed to be dominant in thin (<1 μm) membranes with smooth surfaces up to distances ~0.1–1 mm [31] , [32] , [33] , and in short (<10 μm) 1D beams [34] , as well. Thus, scattering is not expected to destroy coherence in the length scale of the periodicity of our structures (~1–2 μm) if the sidewalls of the holes are smooth, and strong phonon band structure modifications are thus likely to be experimentally observable in thermal transport. The proper geometric design of the PnC, shown in Fig. 1 , was obtained with the help of numerical calculations of the phonon band structure, by solving the 3D elasticity equations for an isotropic material [35] using the finite element method (FEM). Periodic Bloch-wave boundary conditions were used with 2D wave-vectors k in the x – y plane (Methods). 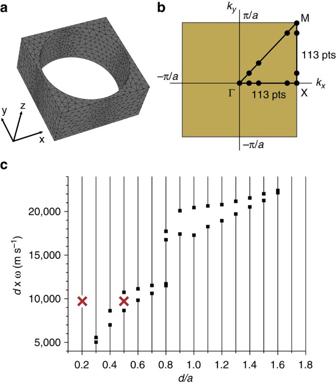Figure 2: Band structure calculations using FEM. (a) A representative unit cell used in the FEM calculations with hole-filling factorf=0.7. A typical mesh structure is also shown. (b) The first BZ of the square PnC lattice ink-space (orange), with the irreducible zone (where calculations are performed) inside the triangle with corners at points Γ,XandM. One typical set of evenly dividedk-points is also indicated. Other, uneven divisions were used, as well. (c) The scaled width of the phononic band gap in SiN (empty region in angular frequencyω) as a function of the ratio of the thickness of the membranedand the lattice constanta. The red crosses show the chosen design values. Figure 2a shows a typical FEM mesh of the unit cell of a perforated square lattice membrane used in the computations. The values of the 2D wave-vector were varied within the irreducible octant of first Brillouin zone (BZ) of a square lattice, shown in Fig. 2b , with a typical number of k -points ~6,400 (the band structure in the rest of the BZs follow from symmetry arguments). Continuous elasticity theory is known to give the correct phonon modes as long as the phonon wavelengths in question are larger than the atomic distances, a condition that is satisfied in the PnC problem from the very outset due to the much reduced size of the BZ compared to an atomic solid (a factor given by the ratio of the PnC period to the atomic lattice period, ~10,000 in our case). Our treatment follows previous phonon band structure calculations in plates [36] , [37] , [38] , but in contrast to earlier work, we had to calculate the band structure to approximately an order of magnitude higher frequencies, to accurately compute the thermal conductance even at 0.1 K. This is because of the fairly significant tail of the thermal phonon population at higher frequencies. For example, to account for 99% of the total energy content in the 2D Debye model at 0.1 K (0.4 K), phonons up to a frequency ~17 GHz (~68 GHz) must be taken into account (the upper limits corresponding to dominant phonons at temperatures 0.5 and 2 K), meaning that several thousand energy eigenvalues had to be computed for each k -vector point. Figure 2: Band structure calculations using FEM. ( a ) A representative unit cell used in the FEM calculations with hole-filling factor f =0.7. A typical mesh structure is also shown. ( b ) The first BZ of the square PnC lattice in k -space (orange), with the irreducible zone (where calculations are performed) inside the triangle with corners at points Γ, X and M . One typical set of evenly divided k -points is also indicated. Other, uneven divisions were used, as well. ( c ) The scaled width of the phononic band gap in SiN (empty region in angular frequency ω ) as a function of the ratio of the thickness of the membrane d and the lattice constant a . The red crosses show the chosen design values. Full size image After fixing the lattice type and the shape of the hole, we still have three free parameters: the lattice constant a , the thickness of the membrane d , and the areal filling factor of holes f =π r 2 / a 2 , where r is the radius of the hole. Previous numerical studies [8] , [39] have shown that complete elastic band gaps are possible to achieve for square lattice circular hole structures near the close packed value f =π/4=0.785. The structural integrity of course gives a limit about how close to close packing one can approach; here, we have chosen the value f =0.7 because it is practically realizable for micron scale periodicity, and yet has shown to produce complete band gaps in the previous numerical studies [8] , [39] . To fix d and a , we calculated band structures as a function of the ratio d / a using the known elasticity parameters for SiN, and studied how the full phononic band gap evolved, shown in Fig. 2c . Interestingly, the band gap has a non-monotonous behaviour as a function of d / a as has been noted before [8] , with a gap opening at d / a =0.2–0.3 and then closing around d / a =0.8, but with a second higher frequency gap opening at the same time and finally closing around d / a =1.6. Thus, neither very thin nor thick perforated membranes have an absolute band gap. The largest relative band gaps Δω/ω appear at around d / a =0.4–0.5, and we choose to use the value d / a =0.5 for this reason as our design guide for the first structure, with a gap centred at dω ≈10,000 m s −1 . To have a strong effect on the thermal transport, we then choose to set the centre of the band gap to the frequency of thermally dominant phonons at 0.1 K in the 2D Debye model, ħ ω dom,2D =1.594 k B T , giving the frequency v = ω /(2π)≈3.3 GHz (the 2D Debye model gives approximately the same dominant frequency as a full calculation with the real Lamb-modes [35] of the uncut membrane). In terms of the dominant wavelength λ dom , 3.3 GHz corresponds to λ dom =2π ν ave / ω dom =1.8 μm with an average speed of sound appropriate for SiN ν ave =5800, m s −1 . Therefore, the thickness of membrane d is set to 485 nm and hence, the lattice constant should be a =2 d =970 nm ≈λ dom /2. With a hole-filling factor f =0.7, this translates into a hole diameter of 916 nm, leaving bridges in between the holes with a neck width of 54 nm. As shown in Fig. 1c , these dimensions were quite accurately fabricated with the help of e-beam lithography (see Methods). The second structure was then chosen to be in a parameter region with a negligible gap and far from the first design by choosing d / a =0.2, but keeping d and f constant. This leads to a design with a lattice constant a =2425, nm and a neck width of 136 nm. Classically [40] (in scattering based models), the two structures are then expected to have the same thermal conductance. Theoretical phonon band structure In Fig. 3 , we compare the dispersion relations of a full, uncut SiN membrane of thickness of d =485 nm with the results for two square lattice PnCs of the same thickness and with the chosen dimensions, shown in the main symmetry directions Γ-X-M-Γ up to frequency v =20 GHz (or angular frequency ω =2π v =120 rad s −1 ). This range contains essentially all (~99%) of the populated phonons at 0.1 K, so that Fig. 3 gives a full picture of all the modes that affect thermal transport at that temperature. For higher temperature results, we calculated eigenvalues up to a frequency of 35 GHz (50 GHz) for the long period (short period) PnC. The full membrane does not have periodicity, and the calculations were performed using the well-known analytical results of Lamb-mode theory [35] , [41] up to v =160 GHz. We have nevertheless plotted the bands in the same square lattice BZ to help with the comparison. In addition, we have also calculated the full membrane dispersions using FEM simulations, finding perfect agreement with the analytical results (taking into account the effect of the folding in the first BZ), and thus demonstrating the sufficient numerical precision of our approach. 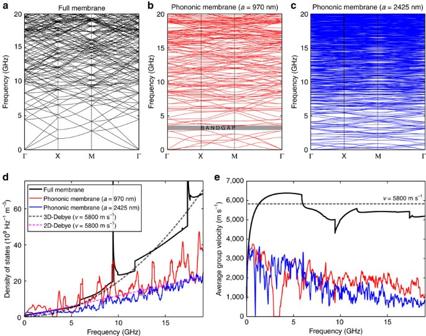Figure 3: Band structure DOS and group velocity. Dispersion relations (band structure) in the main symmetry directions of the BZ for the SiN (a) full membrane (d=485 nm), (b) square lattice PnC, withf=0.7 anda=970 nm, and (c) square lattice PnC, withf=0.7 anda=2425, nm. Complete band gap is observable at 3.3 GHz for the PnC witha=970 nm. (d) The corresponding densities of states (PnCa=970 nm, red, PnCa=2425, nm, blue, full membrane, black) with 2D (pink dash) and 3D (grey dash) Debye models. (e) Average group velocity (averaged over the whole 2D BZ) for full (black) and the two PnC membranes (PnCa=970 nm, red, PnCa=2425, nm, blue). The PnC DOS and group velocity curves have been smoothed for visual clarity. Figure 3: Band structure DOS and group velocity. Dispersion relations (band structure) in the main symmetry directions of the BZ for the SiN ( a ) full membrane ( d =485 nm), ( b ) square lattice PnC, with f =0.7 and a =970 nm, and ( c ) square lattice PnC, with f =0.7 and a =2425, nm. Complete band gap is observable at 3.3 GHz for the PnC with a =970 nm. ( d ) The corresponding densities of states (PnC a =970 nm, red, PnC a =2425, nm, blue, full membrane, black) with 2D (pink dash) and 3D (grey dash) Debye models. ( e ) Average group velocity (averaged over the whole 2D BZ) for full (black) and the two PnC membranes (PnC a =970 nm, red, PnC a =2425, nm, blue). The PnC DOS and group velocity curves have been smoothed for visual clarity. Full size image It is immediately evident that there are great differences between the band structures: the PnC membrane has of course the band gap at frequency 3.3 GHz with a width 0.7 GHz as designed, but this width is still a small fraction of the whole range of frequencies plotted. This implies that the band gap alone has only a minor effect on thermal transport. However, the bands in both PnC structures are also much flatter; this will affect both the group velocities ∂ ω /∂ k and the density of states (DOS), and because both factors influence thermal conductance, one cannot immediately see whether there is a suppression or enhancement. (The thermally transported power is proportional to the product of the DOS and the average group velocity at each energy, weighed by the Planck’s thermal distribution ħ ω /[exp(ħ ω / k B T )−1]). In Fig. 3d , we plot the DOS for both PnC membranes and the full membrane, using the whole calculated dataset (that is, all k -values) up to 19 GHz. The DOS comparison shows a couple of interesting features: (a) In the low-frequency region below ~6 GHz, the full membrane follows the 2D Debye model DOS~ ω , but then starts to grow faster approximately as ~ ω 2 at higher frequencies, roughly in agreement with the 3D Debye model. Thus, 6 GHz is roughly the 2D–3D transition for SiN membranes of thickness 485 nm, where the higher order ‘optical’ Lamb-modes (with finite frequency at k =0) start to contribute. (This transition frequency scales as 1/ d ). (b) On the other hand, the DOS for both PnC membranes follows, on the average, the 2D Debye model all the way up to 19 GHz so that it does not exhibit such a transition, and the DOS above 6 GHz is therefore reduced by an increasingly large factor, up to ~3 at 19 GHz as compared to the full membrane. (c) The fluctuations of the PnC DOS are much larger than in the full membrane, and largest for the smaller period PnC. This is because of the flatness of the bands, leading to many more van Hove singularities. (d) The PnC DOS is higher than the full membrane at frequencies below the band gap at 3.3 GHz for the smaller period structure (below 1 GHz for the larger period PnC), at certain frequencies by a factor of ~2. This will play an important role in the heat conduction, as will be discussed below. An example of the effect of the PnC on the group velocities, on the other hand, is shown in Fig. 3e . Average group velocities are much smaller in the PnC membranes, by a factor up to six at frequencies above 15 GHz, and by a factor of ~2 just below the band gap at 3.3 GHz. In conclusion, based on the DOS and group velocity changes, one definitely expects a suppression of thermal conductance for both PnC structures at T >0.1 K, and the strength of the suppression is expected to grow as temperature increases. At very low frequencies and thus temperatures, the effects of the group velocity and DOS reductions are small so that the PnC thermal conductance is expected to approach the full membrane result. Thermal conductance experiment and comparison to theory The heat conduction experiments on both PnC devices were performed by applying a known power (up to a few nW) electrically at the centre of the device, and by measuring the resulting phonon temperature rise, as in refs 26 , 34 , 42 . This was achieved by employing Al-AlOx-Cu-AlOx-Al superconductor/insulator/normal metal/insulator/superconductor (SINIS) tunnel junction pairs ( Fig. 1d ) both as a thermometer [24] , [26] , [43] and a heater [42] , [44] mounted at the centre of the PnC, with the bath temperature kept below 0.1 K using a dilution refrigerator (Methods). The main benefit of using tunnel junctions here is that both the temperature measurement and the heat dissipation are localized at the centre of the membrane, providing a fairly idealized setting for two-dimensional non-directional heat flow. In addition, the self-heating power in the thermometer is so small (<0.2 pW in all experiments here) that sub-pW range phonon emission power can be measured. For comparison, the experiments were also repeated on uncut, full membrane devices with otherwise exactly the same device fabrication details. The dependence of the measured emitted power P versus measured membrane temperature for both PnC samples and the full membrane are shown in Fig. 4 , up to about 1 K. One clearly sees that the emitted power is much reduced for both PnC membranes at all temperatures, compared to the full membrane result. Unintuitively, the larger period PnC actually has a lower thermal conductance than the smaller period structure, which has the maximal band gap. Clearly, maximizing the band gap does not necessarily lead to minimum thermal conductance. Interestingly, the reduction factor is also strongly dependent on the temperature: at the low-temperature end of the experiment ~0.2 K, the larger period (smaller period) PnC conducts about 14 (5) times less, but at the higher end T ~0.5 K, this reduction has grown to factors ~30 (8). Clearly, the temperature dependence of conductance is quite different in the full membrane and PnC cases, with approximate dependencies P ~ T 3.3 and P ~ T 2.3 at low T for the full and PnC membranes, respectively, whereas closer to 1 K both the full membrane and the short period PnC samples have P ~ T 4 and the long period PnC closer to P ~ T 5 . 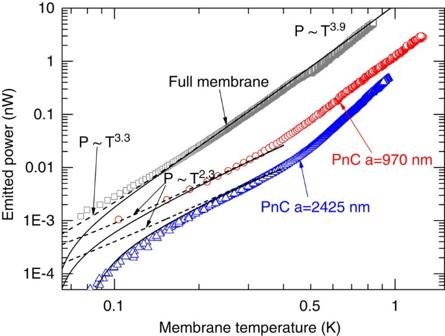Figure 4: Measured emitted phonon power versus temperature. Grey squares show the data for the full, uncut membrane, red circles (a=970 nm) and blue triangles (a=2425, nm) the data for the two square PnC samples. The theoretical lines are given by Equation (1), using the computed band structures for each case, with (solid lines) or without (dashed lines) a phonon back radiation power from the substrate at bath temperature (60 mK for full membrane and PnC witha=970 nm, 80 mK for PnC witha=2425, nm). All three theory curves were fitted to the data with one common scale parameter. The size of symbols represent measurement errors. Figure 4: Measured emitted phonon power versus temperature. Grey squares show the data for the full, uncut membrane, red circles ( a =970 nm) and blue triangles ( a =2425, nm) the data for the two square PnC samples. The theoretical lines are given by Equation (1), using the computed band structures for each case, with (solid lines) or without (dashed lines) a phonon back radiation power from the substrate at bath temperature (60 mK for full membrane and PnC with a =970 nm, 80 mK for PnC with a =2425, nm). All three theory curves were fitted to the data with one common scale parameter. The size of symbols represent measurement errors. Full size image This strong difference in the temperature dependence between the full membrane and the two PnC samples rules out the possibility that thermal conductance in our experiments would be limited by diffusive scattering inside bulk SiN, because in that case the temperature dependences of all the samples should be the same with a constant reduction factor in thermal conductance between the full membrane and both PnC samples, given simply by the geometrical filling factor-dependent effect due to the holes [40] . In addition, if diffusive surface scattering at the hole edges dominated [45] , the longer period PnC sample should produce a higher and not a lower thermal conductance, as the neck dimensions are larger but the edge roughness the same. In terms of thermal conductance defined as G = P /Δ T , where Δ T = T meas − T bath , G ~6 pW K −1 , ~30 pW K −1 , and ~80 pW K −1 for the larger period PnC, smaller period PnC and full membrane, respectively, at 0.1 K. Thus, PnC devices offer a way to reduce thermal conduction by a significant factor, without having to reduce the membrane thickness. We can also understand the observations in a quantitative manner. We have therefore calculated the ballistic phonon power emitted from a convex heater surface γ perpendicular to the membrane surfaces ( Fig. 1a ), without taking into account the acoustic mismatch between the PnC and the unmodified membrane in the vicinity of the heater, or the mismatch at the membrane-bulk edge. For an unmodified 2D membrane, this was already discussed in refs 46 , 47 using the well-known Rayleigh-Lamb modes of suspended membranes [35] , [48] . Here, we extend the calculations to PnC membranes, for which the radiated power is given by where ω j ( k ) is the calculated PnC band structure in the first 2D BZ K , n (ω j , T ) is Bose–Einstein distribution, and only positive group velocities ∂ ω j /∂ k with respect to the heater boundary surface normal contribute to the emitted power, taken into account by the step function Θ. Note that for a large, dense set of eigensurfaces (here we calculated up to ~2,400 2D ω j ( k ) surfaces), errors are generated in the group velocity calculations around the surface intersections, if the eigensurfaces are simply sorted by increasing ω (as is usually the output of FEM solvers). We have developed an algorithm [49] (Methods), which sorts the eigensurfaces according to their real mode structure, so that correct group velocities and thus correct phonon emission power can be calculated. The theoretical calculations for P ( T ) are also shown in Fig. 4 as solid and dashed lines, where the solid lines take into account phonon back radiation from the substrate at the bath temperature, and dashed lines do not. Note that only one common scale factor for P is used in fitting all three experimental curves. We observe that the agreement with the measured temperature dependences is very good, all the way up to the highest temperatures calculated, which for the full membrane could be extended all the way up to 1 K with the help of the analytical dispersion relations, and for the PnC membranes up to ~0.4 K, limited by the computing resources available. The full membrane data seems to follow the theory without back radiation better at very low temperatures, a fact which we cannot currently explain. As the heater dimensions were the same for all samples, the theory also predicts how much in absolute terms the power should be reduced between the ideal membrane and the PnC samples. Clearly, the data agrees almost perfectly with the predicted reduction, giving us further strong evidence that the thermal conductance is governed solely by the coherent band structure modifications and not by scattering, at least below 0.4 K. Finally, to gain some further physical understanding on why the PnC thermal conductance is less suppressed at low temperatures, we have calculated the emitted spectral powers P ( v ), where P = ∫P ( v ) dv , for both full and PnC membranes at two example temperatures T =0.1 K and T =0.3 K, shown in Fig. 5 . As we see, the ints for the PnC devices are smaller than that for the full membrane, consistent with the reduction of total power, and the full membrane results somewhat resemble simple Debye model spectra. The PnC spectral powers are clearly more suppressed at 0.3 K because both the reduced group velocity and the reduced DOS above the band gap have large weight. On the other hand, at 0.1 K more power is carried at lower frequencies, where the DOS is actually enhanced for the PnC, leading to a smaller suppression, as observed in the experiment. 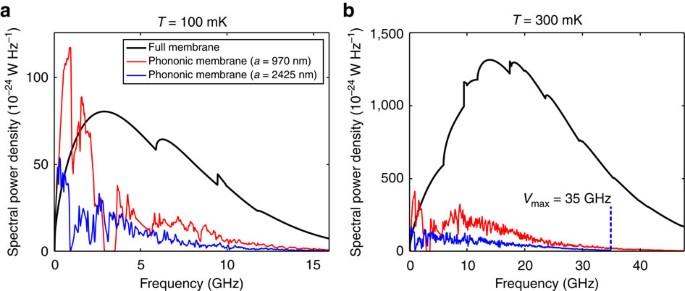Figure 5: The spectral phonon power. We compare the spectral powersP(v) of a full membrane (black line) to the PnC devices (a=970 nm, red line,a=2425, nm, blue line), at (a)T=0.1 K, and (b)T=0.3 K. For thea=2425, nm structure, power was calculated up to 35 GHz. Figure 5: The spectral phonon power. We compare the spectral powers P ( v ) of a full membrane (black line) to the PnC devices ( a =970 nm, red line, a =2425, nm, blue line), at ( a ) T =0.1 K, and ( b ) T =0.3 K. For the a =2425, nm structure, power was calculated up to 35 GHz. Full size image In summary, we have measured the thermal conductance G of two-dimensional PnCs at sub-Kelvin temperature range for the first time. The results are consistent with the picture that phonon transport in the PnC is strongly suppressed by the coherent modification of the phonon band structure caused by the periodic hole structure. The main influence to thermal conductance comes not from the existence of a band gap directly, but from the combination of the reduction of the group velocities and the DOS, leading to a strong reduction of G by over an order of magnitude. However, at the lowest frequencies, the PnC DOS can actually be enhanced, leading to a smaller reduction at the lowest temperatures measured ~0.1 K. As the temperature dependence and the magnitude of thermal conductance are both modified and fully consistent with the theoretical band structure calculations, we have evidence that the reduction of G is not a simple geometrical effect on bulk or boundary scattering limited thermal conductivity. Our results therefore imply that it is possible to lower G significantly without having to sacrifice the mechanical robustness of a thicker membrane or without having to resort to the more delicate beam geometry, facts that might be useful directly in some cryogenic detector devices. Our results also give a model picture of what the theoretical limits are at higher temperatures, if scattering effects were minimized and dimensions properly scaled. In fact, as a large proportion of heat, even at room temperature, is carried by phonons with relatively long mean free paths >1 μm [50] , [51] , [52] , our results may have relevance to room temperature thermal transport, as well. In the future, the role of different lattice structures, shape of the holes and other design factors should be investigated further. Device fabrication The samples were fabricated on single crystal (100) Si wafers with double-sided 750 nm thick low-stress SiN films grown by low-pressure chemical vapour deposition and purchased from the Microfabrication Laboratory at UC Berkeley. To obtain membranes of thickness d =485 nm, the chips were etched from the top side by reactive ion etching (RIE) (Oxford Instruments Plasmalab 80) in CHF 3 /O 2 gas mixture (10:1) with a low power of 50 W, which was effective to keep the surface roughness low at ~0.3 nm (RMS). The obtained thickness was measured using both an ellipsometer (Rudolph AutoEL III) and a thickness profiler (KLA Tencor P-15). The RIE thinning etch was followed by a photolithography step, where a ~625 μm × 625 μm square was patterned and etched through the bottom-side nitride, using again RIE in CHF 3 gas. The remaining backside SiN then served as an etch mask for a crystallographic potassium hydroxide (KOH) wet etch through the whole Si wafer thickness (300 μm), producing a 485 nm thick suspended SiN membrane of size ~200 μm × 200 μm on the front side (bulk micromachining). The tunnel junction heater and thermometer were fabricated next on the membrane. The metal wire structures were deposited using electron-beam lithography and two-angle shadow mask technique, where the the two metals aluminium (Al) and copper (Cu) were electron-beam evaporated from different angles in an UHV system with a base pressure 10 −8 mbar. The angle evaporation was made possible by a two-layer resist (PMMA/MMA-MAA) that formed a large undercut structure. Al was evaporated first to a thickness 16 nm (speed 0.2 nm s −1 ) from 60° angle with respect to the normal of the substrate, after which it was thermally oxidised in situ in 100 mbar for 4 min, producing a thin AlOx barrier. Then, Cu was evaporated to a thickness 40 nm with rate 0.15 nm s −1 from 0° angle, which produced the desired Al/AlOx/Cu/AlOx/Al SINIS tunnel junction structures after the lift-off, as shown in Fig. 1d , with junction dimensions 400 nm × 440 nm and a normal metal island length 10 μm. The junctions with this fabrication sequence typically had a tunnelling resistance R T ~20–40 kΩ. For some samples, a thin 10 nm layer of gold was evaporated on top of Cu to passivate the surface. Finally, to obtain the PnC membranes, a square array of periodic holes of either diameter D =916 nm and period a =970 nm, or D =2290, nm and a =2425, nm were patterned on the membrane by a second round of electron-beam lithography and RIE in CHF 3 /O 2 (10:1) (55 mTorr, 100 W, 26 min) through the membrane, with a 0.9–1.5 μm thick PMMA as the etch mask. The whole perforated region was 100 μm × 100 μm, which translates into 100 (40) periods in both x and y directions for the smaller (larger) period sample. The hole-filling factor 0.7 thus demanded that the narrowest neck widths are <60 (136) nm ( Fig. 1c ). The full membrane fabrication was identical, except that the final perforation etching steps were skipped. Thermal transport measurement All measurements were perfomed in a 3 He– 4 He dilution refrigerator with a base temperature of ~60 mK with several stages of filtering in the wires, because of the extreme sensitivity of the tunnel junction devices to unwanted spurious power loads. Care was taken to filter out unwanted external RF noise from the experiment to <1 pW. The setup uses shielded coax wiring from room temperature to 4 K flange, where a RC-filter stage is located. From 4 K to 60 mK, the wires are Thermocoax cables of length ~1.5 m, with known good attenuation properties at high frequencies [53] . In addition, another set of RC-filters are located at the 60 mK sample stage, inside a copper box thermalized to T bath . In the experiment, the temperature of one SINIS tunnel junction thermometer was measured as a function of the bias voltage across the second SINIS device, used as a heater. The dissipated power in the heater was measured by measuring simultaneously both the current with a current preamplifier (Ithaco 1211) and the voltage across the heater with a high input impedance differential voltage preamplifier (Ithaco 1201). Note that all the leads are superconducting Al, thus all dissipation takes place at the junctions in the middle of the membrane, and the heat flow geometry is two-dimensional. The effect of the temperature drop between the heater and the thermometer was kept constant in all experiments by keeping the size of the heater and the thermometer and the distance between them constant. The bias voltages on the heater are, on the other hand, high enough that the superconducting gap does not influence the heat dissipation at the junctions, and the junctions behave effectively as normal-insulator-normal junctions. The second SINIS junction pair was used as a sensitive thermometer because of their highly non-linear and temperature-dependent current–voltage (I–V) characteristics at sub-Kelvin temperatures [24] , [26] , [43] . In practice, the measurement is usually performed in a constant current bias mode by measuring the temperature-dependent voltage response. When current biased, the SINIS thermometer voltage is a sensitive function of temperature only, and this dependence is typically fully understood by the single-particle tunnelling theory [24] , [26] , [43] with all parameters (tunnelling resistance of the junctions R T , the superconducting gap Δ and the effective broadening of the superconducting DOS) determined self-consistently from the current–voltage curves of the junctions ( Fig. 6a ). In practice, we always performed a calibration measurement, where the measured SINIS voltage was compared with the bath temperature given by a calibrated RuO thermometer while the refrigerator temperature was varied, without the electrical heating of the heater junctions ( Fig. 6b ). This way, any possible non-equilibrium effects (where electron temperature of the devices differs from the lattice temperature) due to the junction bias and external heat loads are self-consistently corrected for. 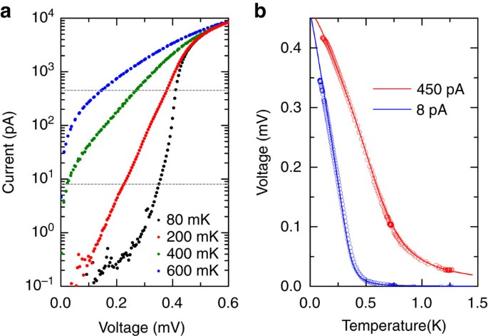Figure 6: Superconducting tunnel junction thermometer characteristics. (a) Measured subgap current–voltage characteristics of a typical superconductor-insulator-normal metal-insulator-superconductor (SINIS) thermometer (2RT=43 kΩ) at different bath temperatures in log-linear scale. Horizontal dashed lines correspond to bias currents 450 pA and 8 pA. (b) Measured voltage-bath temperature response of the SINIS thermometer in (a) with two different values of bias current, 8 pA (blue circles) and 450 pA (red circles) (same values as the lines in (a)). Solid lines were calculated using the single-particle tunneling theory, Equation 2. Bath temperature was measured with a calibrated RuO thermometer. The upper limit for a SINIS thermometer is set by the critical temperature of the superconductor, which means that for Al structures it can operate up to ~1 K. Figure 6: Superconducting tunnel junction thermometer characteristics. ( a ) Measured subgap current–voltage characteristics of a typical superconductor-insulator-normal metal-insulator-superconductor (SINIS) thermometer (2 R T =43 kΩ) at different bath temperatures in log-linear scale. Horizontal dashed lines correspond to bias currents 450 pA and 8 pA. ( b ) Measured voltage-bath temperature response of the SINIS thermometer in ( a ) with two different values of bias current, 8 pA (blue circles) and 450 pA (red circles) (same values as the lines in ( a )). Solid lines were calculated using the single-particle tunneling theory, Equation 2. Bath temperature was measured with a calibrated RuO thermometer. Full size image The thermometer junctions were current biased with a bias resistor R =1–10 GΩ to ensure proper current bias even in the subgap, where junction resistance was typically ~1–10 MΩ at low temperatures. In the experiment, two different constant bias current values ( I ~10 pA) and ( I ~500 pA) were typically used, the low one for low-temperature regime T <0.4 K and higher one for high-temperature regime T >0.4 K. Two values were used because the SINIS temperature-to-voltage responsivity dV / dT is a strong function of both I and T in such a way that the low-bias (high-bias) value gives a better responsivity at T <0.4 K ( T >0.4 K), see Figure 6b . In addition, the lower bias value was always chosen higher than the measured two-electron/life time-broadened excess subgap current (observable below 1 pA in Fig. 6a ), to guarantee good response and no dependence on the details of the excess current mechanisms. The thermometer voltage was measured with a high input impedance differential voltage preamplifier (Ithaco 1201). The I–V and V–T characteristics can be understood by a simple tunnelling Hamiltonian theory [24] , [54] , which predicts for a pair of identical normal metal-superconductor tunnel junctions connected in series (SINIS) where R T is the tunnelling resistance of a single junction, f N ( E ) is the Fermi-function of the normal metal in quasiequilibrium and g S ( E ) is the quasiparticle DOS in the superconductor. Note that equation (2) contains only the temperature of the normal metal and not that of the superconductor, and is valid as long as the quasiparticle distribution in the superconductor is also in quasiequilibrium (but not necessarily the same temperature). g S ( E ) can be determined from the Bardeen–Cooper–Schrieffer theory, which predicts in the weak coupling limit that , when | E |>Δ and g S ( E )=0 when | E |<Δ (ref. 54 ). However, in real materials there are processes that create quasiparticle states also within the gap | E |<Δ. The easiest and most straightforward way to model these is with the so called Dynes-parameter, which was initially realized to model life time broadening due to inelastic scattering (electron–electron, electron–phonon) [55] . This leads to a DOS of the form where parameter Γ described originally the finite life time of quasiparticle states in the superconductor. However, it was recently shown [56] that exactly the same model follows from the theory of environmentally photon-assisted tunnelling processes, as well, and that therefore, the parameter Γ is not necessarily a materials parameter, but depends on the degree of filtering out unwanted microwave photons. In our devices, the Dynes model always fits the deep subgap I–V characteristics well (current below ~1 pA in Fig. 6a ), and its value simply sets the minimum bias current for thermometer operation, below which the temperature responsivity goes to zero. Details on finite element method simulations The phonon frequency spectrum ω j ( k ) was numerically calculated by the FEM (Comsol Multiphysics v4.1 software) from the elastic Lamé system for the 3D displacement vector u in the unit cell Ω of the periodic membrane, which in our case, is a single circular hole inside a square, see Fig. 2a . μ, λ and ρ are the material-dependent elastic parameters and density, respectively. The boundary conditions in Equation 4 describe the stress free condition at the inside hole wall and the membrane top and bottom surfaces, where σ( u ) is the stress tensor and the surface normal, and also Bloch’s theorem conditions at the boundaries connecting the unit cells. Typical unit cell was divided into a mesh with up to ~22,000 elements, with a denser mesh around the narrower regions ( Fig. 2a ). μ and λ are connected with the experimentally measurable parameters Young’s modulus E and Poisson’s ratio v , by the relations λ= Ev /[(1+ v )(1−2 v )], μ= E /[2(1+ v )]. In the simulations, we have used the values E =250 GPa, v =0.23 and ρ=3,100 kg m −3 for amorphous SiN [57] . Bloch’s theorem guarantees the existence of plane wave-type solutions u j ( x , y , z ; k ) with eigenfrequencies ω j ( k ). The FEM eigenvalue algorithm organizes the eigenfrequencies ω j ( k ) to an increasing order for each k , defining continuous energy surfaces for j =1,…, N . However, using the raw set of eigenfrequencies causes a systematic error in the calculated group velocities near the intersections of the surfaces, because these unsorted surfaces do not necessarily correspond ‘to the same’ phonon mode for two distinct k i ≈ k j near the intersection, see Fig. 7 . This gives rise to an error in the total radiated power, which increases at high temperatures, as the number of branch intersections increases with the increasing DOS. In Fig. 7c we show as an example the relative error in P ( T ) for various k -space grid densities of a non-perforated (solid) membrane with d =485 nm. For this case, the group velocities can also be calculated analytically from the Rayleigh-Lamb equations [35] , therefore, we know exactly what the error is. It can be seen that the relative error can be sizeable at temperatures above 100 mK, and cannot be controlled easily by just increasing the number of k -space grid points. Therefore, we have developed an algorithm [49] , which correctly identifies how the eigensurfaces continue across intersecting lines, as shown in Fig. 7b . 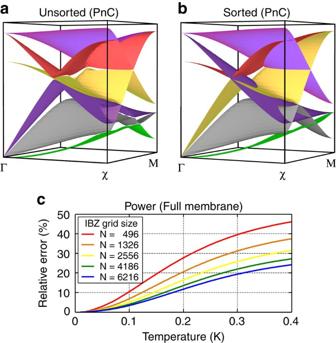Figure 7: Sorting of eigensurfaces. Low energy spectral branches of a 2D PnC with circular hole perforations plotted over the irreducible BZ (IBZ). (a) Unsorted surfaces, which provide incorrect group velocity data atk-values where the surfaces intersect. (b) Sorted surfaces, which correspond to the eigenmodes continuous ink. (c) Relative error inP(T) for a full membrane withd=485 nm for various IBZ grid sizes, when eigensurface sorting is neglected. Eigensurfaces were calculated up to 70 GHz. Figure 7: Sorting of eigensurfaces. Low energy spectral branches of a 2D PnC with circular hole perforations plotted over the irreducible BZ (IBZ). ( a ) Unsorted surfaces , which provide incorrect group velocity data at k -values where the surfaces intersect. ( b ) Sorted surfaces, which correspond to the eigenmodes continuous in k . ( c ) Relative error in P ( T ) for a full membrane with d =485 nm for various IBZ grid sizes, when eigensurface sorting is neglected. Eigensurfaces were calculated up to 70 GHz. Full size image Even with sorted eigensurfaces, one can still have numerical error in the computation owing simply to lack of higher energy eigensurfaces. We estimate that at the highest temperatures calculated here for the PnC structures (0.4 K), the error introduced by the upper bound in frequency range (35 GHz for the long period PnC and 50 GHz for the short period PnC) is the dominant one, of the order of at least several tens of per cent. How to cite this article: Zen, N. et al. Engineering thermal conductance using a two-dimensional phononic crystal. Nat. Commun. 5:3435 doi: 10.1038/ncomms4435 (2014).